Free-decay and resonant methods for investigating the fundamental limit of superhydrophobicity The recently demonstrated extremely water-repellent surfaces with contact angles close to 180° with nearly zero hysteresis approach the fundamental limit of non-wetting. The measurement of the small but non-zero energy dissipation of a droplet moving on such a surface is not feasible with the contemporary methods, although it would be needed for optimized technological applications related to dirt repellency, microfluidics and functional surfaces. Here we show that magnetically controlled freely decaying and resonant oscillations of water droplets doped with superparamagnetic nanoparticles allow quantification of the energy dissipation as a function of normal force. Two dissipative forces are identified at a precision of ~ 10 nN, one related to contact angle hysteresis near the three-phase contact line and the other to viscous dissipation near the droplet–solid interface. The method is adaptable to common optical goniometers and facilitates systematic and quantitative investigations of dynamical superhydrophobicity, defects and inhomogeneities on extremely superhydrophobic surfaces. Non-wetting surfaces have experienced an enormous boost of interest [1] , [2] , [3] , [4] after the observation of superhydrophobicity and self-cleaning effect in natural lotus leaves [5] . Artificial superhydrophobic coatings have been developed and used in self-cleaning [5] , [6] , antifogging [7] and anti-icing [8] materials, non-wetting textiles [9] , heat-transfer interfaces [10] , drag-reducing coatings [11] , and for storing and displaying information [12] . Generally, superhydrophobicity arises from a combination of surface roughness and a low-energy coating [6] . Many intriguing properties of superhydrophobicity originate from the metastable Cassie-Baxter state in which water droplets rest partly on air that is trapped within the nano- and microstructures of the rough surface [13] , [14] . Liquid flowing partly over the trapped air exhibits macroscopic viscous slip, that is, non-zero flow at the apparent solid–liquid boundary [15] . The slip can reduce viscous drag [16] , [17] and thus enhance flow in micro- and nanochannels [15] as well as in sessile droplets [19] , [20] , [21] . Combining the reduced drag with the guidance of the droplets by gravitational [18] , electric [18] or magnetic fields [19] , [20] opens platforms for novel functional droplet devices performing, for example, logic operations or programmable chemistry [21] . Many applications of superhydrophobicity rely on accurate understanding of how the kinetic energy is dissipated by droplets moving on these non-wetting surfaces. Whereas the slip and viscous drag reduction have been extensively characterized in continuous flows by, for example, nanorheological measurements [22] and particle image velocimetry [23] , considerably less is known about the friction and dissipation in discrete droplets. This can be considered to originate from the contemporary characterization methods, such as the optical contact angle goniometry, that measure static or quasi-static properties of the interfaces and contact angles [24] . The quasi-static measurements can yield only indirect information of some of the dissipative processes, such as the contact angle hysteresis (CAH) force caused by e.g. surface heterogeneity. Moreover, those measurements are severely hindered by optical errors when approaching the fundamental limit of non-wetting, that is, advancing and receding contact angles of 180° (ref. 25 ). Further complications arise from the time-dependent nature of the contact angles of static droplets [26] , [27] . Dissipation in actual moving droplets has been investigated by observing gravitation-induced droplet motion on tilted superhydrophobic substrates [27] , [28] , [29] . However, the method suffers from the inability to control the normal and lateral forces independently. This is a major drawback because the relationship between these forces can be non-trivial [30] , [31] . A centrifugal adhesion balance can overcome the force coupling problem, but is more suitable for quasi-static measurements (for example, to study the lateral force required to unpin a droplet) than for dynamic measurements (for example, to investigate energy dissipation and the corresponding dissipative forces as a function of droplet speed). Moreover, surface defects and surface inhomogeneity are challenging to probe by using any of the conventional methods. Thus, new approaches are needed for studying directly the energy dissipation in dynamic moving droplets under well-defined lateral and normal forces, in order to understand energy dissipation, defects and wear on the intrinsically fragile superhydrophobic surfaces [32] . On a general level, oscillatory concepts are often preferred in measurement technologies [33] . They are especially suitable for studying systems with minimal energy dissipation, for example through gradually decaying free oscillations or through the linewidths of externally driven resonance peaks. These approaches allow probing the dissipation with inverse sensitivity, i.e. the accuracy increases with decreasing dissipation. In this work, we present a method for measuring kinetic energy dissipation by observing the transverse oscillating motion of droplets on superhydrophobic surfaces under well-controlled normal and lateral forces. The method is based on dispersing a small amount of magnetic iron oxide nanoparticles in water, which allows any combination of forces to be exerted on the droplet through an external non-uniform magnetic field. We show that both freely decaying and externally driven resonant harmonic oscillations can be generated by confining the droplet in a harmonic magnetic potential well. The damping rate of the freely decaying oscillations and the linewidth of the resonance yield quantitative values for the CAH and viscous forces at a precision of ~ 10 nN. We apply the oscillatory method for establishing the scaling relationships between the dissipative and normal forces experimentally for the first time. Oscillating magnetic droplet in a harmonic potential well We first used an extremely superhydrophobic surface based on a self-assembled monolayer of a fluorinated surfactant covering a rough nanosilver coating [2] as a test surface for our oscillatory methods. A harmonic potential well was realized on the superhydrophobic surface by placing an axially magnetized cylindrical permanent magnet under or above the test surface ( Fig. 1a ). The resulting magnetic field H has the spatial dependency of H = H 0 – cx 2 /2, where x is the distance from the centre of the potential well (axis of the magnet), H 0 the field strength on the axis and c> 0 the steepness of the potential well (field curvature). The field strength and curvature can be conveniently adjusted by changing the distance between the magnet and the substrate or by using differently sized magnets ( Supplementary Fig. S1 ). The magnetic potential energy of the droplet, U =− μ 0 HMV , where M is magnetization and V is volume of the droplet, increases when the droplet is displaced from the symmetry axis ( Fig. 1b ). As a result, a displaced droplet experiences a Hookean restoring force , where . This force brings the droplet into an oscillatory motion that is damped by the dissipative forces ( Fig. 1c and Supplementary Movie 1 ). As shown in the following, the dissipative forces ( Fig. 1d ) can be determined from the rate at which these oscillations decay. 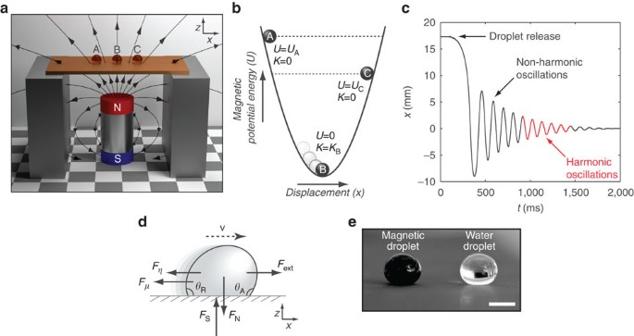Figure 1: A magnetic water droplet in a harmonic potential well. (a) A schematic 3D rendering of the experimental set-up for creating a harmonic magnetic potential well on a superhydrophobic substrate by placing a cylindrical permanent magnet below (or above, not shown) the substrate. The droplet is shown in three positions: extreme left (A), centre (B) and extreme right (C). (b) A schematic figure of the harmonic potential well with the droplet shown in three positions as in figure (a). The total energy of the dropletE=U+K(sum of magnetic potential energyUand kinetic energyK) decreases due to the dissipation as the droplet moves from position A to B and to C, that is,EA>EB>EC. After reaching position C, the motion of the droplet is reversed. (c) The position of the oscillating droplet as a function of time after releasing it. The first few oscillations are discarded from the automated analysis because the harmonic approximation is valid only at small displacements. The last few oscillations are discarded because of the increased probability of pinning of the droplet in defects at small velocities. (d) The force diagram of the magnetic droplet moving at a velocityvto the right, showing the viscous forceFμ, the CAH forceFμand the external magnetic restoring forceFext. The normal forceFNis magnetically adjustable and is equal in magnitude as the support force from the substrateFS, but opposite in sign. The anglesθAandθRdenote the advancing and receding contact angles, respectively. (e) A photograph of a magnetic droplet and a water droplet (both 10 μl) on the extremely superhydrophobic test surface. Scale bar, 2 mm. Figure 1: A magnetic water droplet in a harmonic potential well. ( a ) A schematic 3D rendering of the experimental set-up for creating a harmonic magnetic potential well on a superhydrophobic substrate by placing a cylindrical permanent magnet below (or above, not shown) the substrate. The droplet is shown in three positions: extreme left (A), centre (B) and extreme right (C). ( b ) A schematic figure of the harmonic potential well with the droplet shown in three positions as in figure ( a ). The total energy of the droplet E = U + K (sum of magnetic potential energy U and kinetic energy K ) decreases due to the dissipation as the droplet moves from position A to B and to C, that is, E A > E B > E C . After reaching position C, the motion of the droplet is reversed. ( c ) The position of the oscillating droplet as a function of time after releasing it. The first few oscillations are discarded from the automated analysis because the harmonic approximation is valid only at small displacements. The last few oscillations are discarded because of the increased probability of pinning of the droplet in defects at small velocities. ( d ) The force diagram of the magnetic droplet moving at a velocity v to the right, showing the viscous force F μ , the CAH force F μ and the external magnetic restoring force F ext . The normal force F N is magnetically adjustable and is equal in magnitude as the support force from the substrate F S , but opposite in sign. The angles θ A and θ R denote the advancing and receding contact angles, respectively. ( e ) A photograph of a magnetic droplet and a water droplet (both 10 μl) on the extremely superhydrophobic test surface. Scale bar, 2 mm. Full size image To obtain results that reflect dissipation in pure water droplets, the magnetic fluid should have surface tension γ , viscosity η and density ρ close to those of water. In addition, the magnetic hysteresis losses should be small compared to the energy dissipation due to the frictional forces. We fulfilled these requirements by using a low concentration (0.2% in volume) of superparamagnetic iron oxide nanoparticles stabilized by electrostatic forces in water. The low concentration ensures that the density and viscosity are not markedly changed by the presence of nanoparticles. We confirmed this by direct measurements that showed that η and ρ deviated no more than 4% and 0.7%, respectively, from those of pure water ( Supplementary Fig. S2 ). In addition, the electrostatic stabilization ensures that the surface tension is not changed, which would not be the case if surfactants were used as stabilizers. Indeed, the surface tension of the magnetic fluid was found to be equal to that of pure water ( Supplementary Fig. S2 ). The superparamagnetic nature of the nanoparticles renders the magnetic hysteresis losses negligible, which was confirmed by AC magnetometry ( Supplementary Fig. S3 ). A direct visual comparison between equally sized magnetic and pure water droplets on a superhydrophobic surface also showed similar behaviour in terms of droplet shape ( Fig. 1e ), contact angles and the ability of the droplet to roll off the surface. Kinetic energy dissipation in freely decaying oscillations Typical freely decaying oscillations of a 5-μl magnetic droplet on the test surface are shown in Fig. 2a . Multiple repetitions on the same spot on the test surface showed only a small variation in the droplet motion, indicating high intrinsic precision of the method ( Fig. 2a , upper inset). The potential energy U and the kinetic energy K = mv 2 /2 of the droplet were extracted from the droplet position x ( t ) measured from high-speed (1,000 fps) videos ( Fig. 2b ). Typically, an initial potential energy of ~ 10 nJ at a 3-mm displacement from the symmetry axis of the magnet was dissipated in ~ 1.5 s during five full oscillations. The corresponding average dissipative power is ~ 10 nW. 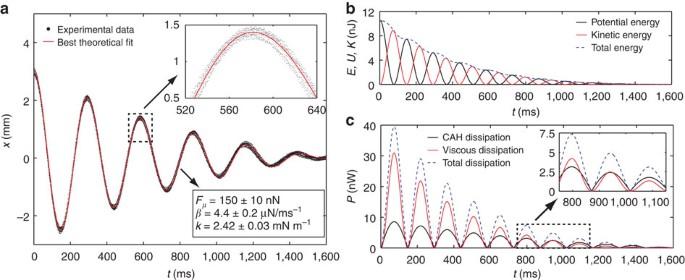Figure 2: Kinetic energy dissipation in freely decaying oscillations. (a) The position (centre of mass of the droplet’s silhouette) of a 5-μl droplet versus time after releasing it from an initial displacement of ~ 20 mm. Measurement was repeated ten times on a single spot on the same superhydrophobic test substrate (seeSupplementary Movie 1). Notice that the first few non-harmonic oscillations are omitted, and only harmonic ones are shown (Fig. 1c). The upper inset shows a close-up of the data for a short time interval, wherein all experimental data points from the ten different measurements can be seen very close to each other. The lower inset shows the parameters extracted from the data by fitting with the analytic solution of the general harmonic oscillator. (b) The corresponding potential energyU, kinetic energyKand total energyE=U+Kas a function of time. (c) The energy dissipation rate and its division into two components due to CAH and viscosity. Figure 2: Kinetic energy dissipation in freely decaying oscillations. ( a ) The position (centre of mass of the droplet’s silhouette) of a 5-μl droplet versus time after releasing it from an initial displacement of ~ 20 mm. Measurement was repeated ten times on a single spot on the same superhydrophobic test substrate (see Supplementary Movie 1 ). Notice that the first few non-harmonic oscillations are omitted, and only harmonic ones are shown ( Fig. 1 c). The upper inset shows a close-up of the data for a short time interval, wherein all experimental data points from the ten different measurements can be seen very close to each other. The lower inset shows the parameters extracted from the data by fitting with the analytic solution of the general harmonic oscillator. ( b ) The corresponding potential energy U , kinetic energy K and total energy E=U+K as a function of time. ( c ) The energy dissipation rate and its division into two components due to CAH and viscosity. Full size image To find out how the dissipation was balanced between CAH and viscosity, x ( t ) was fitted with the solution of the general harmonic oscillator [34] , , where is the viscous force and F μ is the CAH force [34] . The plus sign before F μ applies to v <0 (droplet moving left), negative sign to v >0 (droplet moving right). The fitting yielded values for F η and F μ ( Fig. 2a inset, see Methods for fitting details), based on which the kinetic energy dissipation could be divided into these two contributions ( Fig. 2c ). Both dissipative processes were significant at the measured velocity range (up to 60 mm s −1 ). The viscous dissipation became dominant at velocities above ca. 20 mm s −1 and CAH dissipation at velocities below that. To study surface inhomogeneity, multiple measurements were performed on different spots on the same, seemingly homogeneous superhydrophobic surface. These measurements revealed marked spatial variation in damping of the freely decaying oscillations ( Fig. 3 ). This variation was not due to the measurement technique itself (multiple measurements at any single spot showed much smaller variation, see Figs 2a and 3 ). Thus, the difference in the damping at the two spots was due to the inhomogeneity of the surface itself, proving that even such small variations can be reliably probed with the oscillatory method. 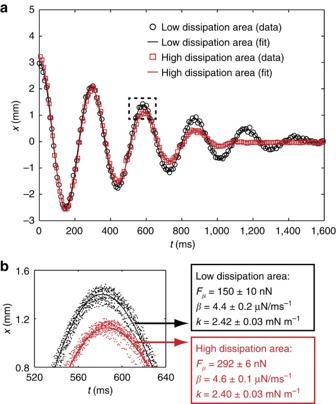Figure 3: Characterization of surface inhomogeneity. (a) The position of a 5-μl droplet versus time measured at two different spots on the same superhydrophobic surface for ten times. (b) Close-up of the data, showing only small variations within the data sets collected at both spots, but a large difference in damping between the two spots. The difference is seen quantitatively in the CAH force that was obtained by fitting the data with the harmonic oscillator model. Figure 3: Characterization of surface inhomogeneity. ( a ) The position of a 5-μl droplet versus time measured at two different spots on the same superhydrophobic surface for ten times. ( b ) Close-up of the data, showing only small variations within the data sets collected at both spots, but a large difference in damping between the two spots. The difference is seen quantitatively in the CAH force that was obtained by fitting the data with the harmonic oscillator model. Full size image The scaling laws between dissipation and normal force No previous study has attempted to establish scaling laws between the kinetic energy dissipation and the normal force. In general, the energy dissipation rate depends on the shape of the droplet near its contact with the surface, which is strongly affected by the normal force ( Fig. 4a ). The length of the three-phase boundary line l and the apparent droplet-surface contact area A both increase with the increasing normal force, as shown by calculations from the Young−Laplace equation ( Fig. 4b ). Here we took advantage of the possibility of using the magnetic field to adjust the normal force on the droplet, which is a sum of the gravitational and the magnetic forces: . Even with small centimetre-sized permanent magnets and nanoparticle concentrations as low as 0.2%, the normal force can be adjusted from g E ≈0 to g E ≈6 g , leading to large changes in the droplet shape ( Fig. 4a,b ). 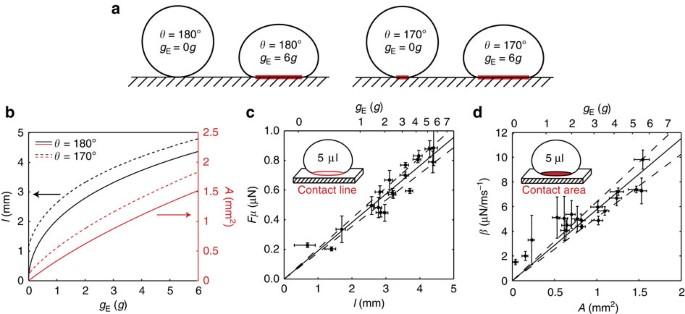Figure 4: Scaling relationship between dissipation and normal force. (a) An illustration of the flattening of a 5-μl sessile droplet upon increasing the normal forcegEfrom 0 to 6 g (calculated from the Young–Laplace equation forθ=170° andθ=180°). (b) The length of the three-phase boundary line and the apparent liquid–solid contact area as a function of the normal force (calculated from the Young−Laplace equation forθ=180° andθ=170°). (c) CAH force as a function of the normal force and the three-phase boundary length, and the best linear fit forced through origin. (d) Viscous dissipation coefficient as a function of the normal force and the apparent area of the liquid–solid interface, and the best linear fit forced through origin. Data in (c,d) were obtained by using several magnetic field strengths, curvatures, vertical gradients and repetitions (Supplementary Fig. S4). Error bars represent standard deviation. Figure 4: Scaling relationship between dissipation and normal force. ( a ) An illustration of the flattening of a 5-μl sessile droplet upon increasing the normal force g E from 0 to 6 g (calculated from the Young–Laplace equation for θ =170° and θ =180°). ( b ) The length of the three-phase boundary line and the apparent liquid–solid contact area as a function of the normal force (calculated from the Young−Laplace equation for θ =180° and θ =170°). ( c ) CAH force as a function of the normal force and the three-phase boundary length, and the best linear fit forced through origin. ( d ) Viscous dissipation coefficient as a function of the normal force and the apparent area of the liquid–solid interface, and the best linear fit forced through origin. Data in ( c , d ) were obtained by using several magnetic field strengths, curvatures, vertical gradients and repetitions ( Supplementary Fig. S4 ). Error bars represent standard deviation. Full size image Freely decaying oscillations performed under this range of normal forces showed a monotonic increase of CAH force with the normal force ( Fig. 4c ). In the first approximation, the increase can be considered to originate from the increasing length of the three-phase boundary line. Thus, the CAH dissipation was fitted with the general expression given by , where the length of the three-phase boundary line l is a function of normal force and is calculated from the Young−Laplace equation [24] , [35] . The best fit was obtained with an average contact angle of θ =176.5±2° and CAH of Δ θ =5±1° ( Fig. 4c ). The ability to capture the dependency of the CAH force on the normal force with single values for contact angle and CAH suggests that these parameters are insensitive to the normal force. The dependency has been much debated [36] , [37] , [38] , [39] , and our results suggest that it may not be necessary to invoke corrections to the contact angles within the normal force range studied here. Instead, the increase in CAH force with the increasing normal force can be explained simply through the increasing length of the three-phase boundary line ( Fig. 4a,b ). The viscous dissipation also increased with the normal force, being nearly linearly proportional to the contact area between the droplet and the surface ( Fig. 4d ). Initially, the observation seems to contradict a model that predicts that a droplet rolling on a perfectly superhydrophobic surface ( θ =180° and Δ θ =0°) should exhibit viscous dissipation proportional to l 3 , that is, the characteristic Hertz volume near the liquid–solid interface [40] . A closer inspection of the surface flows of the oscillating magnetic droplet showed that the droplet does not reach the steady-state rolling motion at any point ( Supplementary Movie 2 ), which is assumed in the model [40] . The droplet moves mainly by sliding, but some rotation can be seen especially in the ends of the half oscillations wherein the droplet momentarily remains almost stationary ( Fig. 5 ). Hence, we hypothesize that the viscous dissipation does not propagate far from the liquid–solid contact area to fill the Hertz volume, and thus becomes proportional to the contact area. Increasing the viscosity of the magnetic droplets by replacing water partially by more viscous ethylene glycol resulted in an increase in β , as expected ( Supplementary Fig. S5 ). 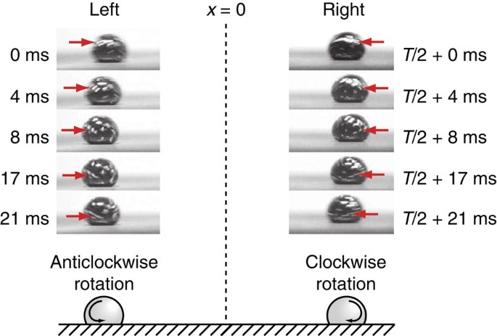Figure 5: Rotation of the droplets in the ends of each half-oscillation. Video frame captures of an oscillating droplet taken at one extreme of the oscillation (left) and subsequently at the other extreme (right) after a half-of-the-periodT/2 (Supplementary Movie 2). The red arrows point to small aluminium particles added to the droplet to help visualize the motion. The motion of the aluminium particles indicates anticlockwise rotation in the left extreme, and clockwise rotation in the right extreme. Figure 5: Rotation of the droplets in the ends of each half-oscillation. Video frame captures of an oscillating droplet taken at one extreme of the oscillation (left) and subsequently at the other extreme (right) after a half-of-the-period T /2 ( Supplementary Movie 2 ). The red arrows point to small aluminium particles added to the droplet to help visualize the motion. The motion of the aluminium particles indicates anticlockwise rotation in the left extreme, and clockwise rotation in the right extreme. Full size image Externally driven resonant measurements The oscillatory method is not limited to investigations of freely decaying oscillations. Resonant measurements can also be implemented. Resonant methods can further increase the precision and allow performing continuous measurements. We realized a simple time-varying external magnetic field by applying a sinusoidal motion to the permanent magnet with angular frequency f and amplitude . The resulting time-varying magnetic force drives an initially stationary droplet to a well-defined forced and continuous oscillation after a transient period ( Fig. 6a ). The final oscillation amplitude of the droplet is dependent on the frequency ( Supplementary Movie 3 ) and a distinct resonance peak was observed near 4.7 Hz ( Fig. 6b ). This corresponds to the resonance of the droplet in the magnetic potential well, the frequency of which depends on the magnetic field curvature and the magnetization of the fluid. At the resonance, the oscillating droplet reached an amplitude of ~ 10 mm, which equals approximately a tenfold amplification of the driving amplitude of 0.9 mm. By fitting the resonance peak shape with the theoretical prediction calculated numerically from the time dependent magnetic force, we obtained once again the CAH and viscous forces in agreement with the results obtained from freely decaying oscillations in a static potential well ( Fig. 6b ). 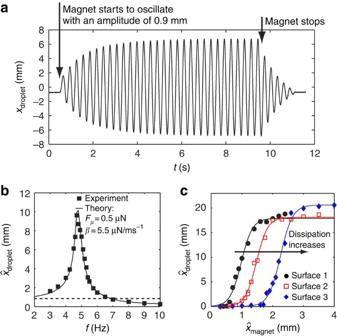Figure 6: Externally driven resonant measurements. (a) Position of the droplet as a function of time after the oscillating magnetic field was turned on (andf=4.7 Hz). The steady-state oscillations were reached after a few tens of oscillations of the magnetic field. After stopping the oscillation, the remaining kinetic and potential energies of the droplet were dissipated by the freely decaying oscillations. (b) The amplitude of the droplet as a function of the frequency of the magnetic field, showing a resonance peak near 4.7 Hz. Dashed line indicates the amplitude of the driving magnet, that is,. (c) Droplet amplitude as a function of the amplitude of the moving magnet for three different superhydrophobic surfaces measured at the resonance frequency (symbols, experiment; lines, sigmoidal fits). Measurements were done on the generic test surface used throughout this manuscript (Surface 1) and on two additional surfaces. Surface 2: fluorinated silicone nanofilaments on a flat SiO2surface (θA=164°,θR=158° and Δθ=6°) and Surface 3: native methyl-terminated silicone nanofilaments on a flat SiO2surface (θA=157°,θR=145° and Δθ=12°). Figure 6: Externally driven resonant measurements. ( a ) Position of the droplet as a function of time after the oscillating magnetic field was turned on ( and f =4.7 Hz). The steady-state oscillations were reached after a few tens of oscillations of the magnetic field. After stopping the oscillation, the remaining kinetic and potential energies of the droplet were dissipated by the freely decaying oscillations. ( b ) The amplitude of the droplet as a function of the frequency of the magnetic field, showing a resonance peak near 4.7 Hz. Dashed line indicates the amplitude of the driving magnet, that is, . ( c ) Droplet amplitude as a function of the amplitude of the moving magnet for three different superhydrophobic surfaces measured at the resonance frequency (symbols, experiment; lines, sigmoidal fits). Measurements were done on the generic test surface used throughout this manuscript (Surface 1) and on two additional surfaces. Surface 2: fluorinated silicone nanofilaments on a flat SiO 2 surface ( θ A =164°, θ R =158° and Δ θ =6°) and Surface 3: native methyl-terminated silicone nanofilaments on a flat SiO 2 surface ( θ A =157°, θ R =145° and Δ θ =12°). Full size image The externally driven measurements are particularly useful for characterization of surfaces with larger CAH, wherein free oscillations would decay too fast. As a demonstration, we studied two additional less superhydrophobic surfaces by observing the droplet amplitude at the resonance frequency as a function of the driving amplitude ( Fig. 6c ). The results showed that the droplets that were initially pinned to the surface due to the CAH were freed when the driving amplitude was increased enough ( Fig. 6c ). The concept of using magnetic droplets for surface characterization opens new possibilities for performing investigations on dynamical superhydrophobicity. The harmonic magnetic potential used in this work is an example among different alternatives, yet very relevant because of the importance of harmonic oscillators in scientific measurements. Investigation of the dissipative forces through the oscillating magnetic droplets produced high-precision quantitative results, as could be expected for oscillatory measurements [33] . Our method not only allows to compare the performances of different superhydrophobic coatings, but also makes it possible to study even the local inhomogeneities and to establish scaling laws between dissipation and normal force. We experimentally showed that in the first approximation the CAH dissipation can be modelled by assuming that the advancing and receding contact angles are independent of the normal force and that the normal force affects the CAH force only by changing the length of the three-phase boundary line. We also demonstrated that low-viscosity droplets that move only short distances exhibit viscous dissipation that is proportional to the contact area between the droplet and the surface. In future, we foresee that the magnetically controlled normal force enables investigation of transitions from the metastable Cassie–Baxter state to the stable high-friction Wenzel state [12] , [41] . The oscillatory method may also serve as an efficient tool for studying the microscopic origins of the wetting dynamics, including the role of the contact line pinning and unpinning that leads to the ‘stick and slip’ behaviour and CAH [42] , [43] . In addition, the demonstrated oscillatory method is compatible with existing optical goniometers and is not limited by the optical errors like in typical goniometric techniques. This suggests that the method holds a promise of becoming a widely used surface characterization tool. The method is especially suitable for studying surfaces close to the fundamental limit of superhydrophobicity, which are challenging to probe with conventional methods. Finally, the ability to use moving droplets in measurements ensures the applicability of the results to real-life droplet transport conditions. Synthesis of iron oxide nanoparticles Iron oxide nanoparticles were synthesized by the coprecipitation method [44] and stabilized by citric acid near pH 7 as described earlier with small modifications [45] . The resulting nanoparticles were dispersed in Milli-Q water with a concentration of Φ =0.2% (volume) and characterized with a transmission electron microscope (JEOL JEM-2200F, 200 kV), yielding an average particle size of 4.6 nm with a geometric standard deviation 1.4 nm ( Supplementary Fig. S3a ). Magnetic properties of the iron oxide nanoparticles The magnetic properties of water containing 0.2% of iron oxide nanoparticles were measured with a SQUID magnetometer (Quantum Design MPMS XL7). Approximately 10 μl of the fluid was placed inside a 3-mm NMR tube, closed with a polypropylene cap and heat-sealed with a heat gun. The NMR tube was placed inside a standard polypropylene straw sample holder for the measurement. The sample holder background was removed using the background subtraction option in the Quantum Design software. The measurements showed hysteresis-free magnetization with a saturation magnetization of 0.8 emu g −1 at 70 kOe. Zero field-cooled and field-cooled curves of the frozen dispersion at 50 Oe were measured, which indicated a broad range of blocking temperatures near 100 K and thus superparamagnetic behaviour at room temperature. Magnetic AC measurements done at similar frequencies as the droplet oscillation measurements further indicated no observable magnetic dissipation. Hence, energy dissipation due to magnetic hysteresis is minimal. For details see Supplementary Fig. S3 . Surface tension of the magnetic fluid Surface tensions of pure Milli-Q water and Milli-Q water containing 0.2% (volume) of iron oxide nanoparticles were measured with the pendant droplet method by using an optical goniometer (Dataphysics OCA20 with 1.65-mm-outer-diameter Nordson Precision Tip 7018062 needles). Images of the pendant droplet were taken for 1 min at the rate of one image per second. Surface tension was obtained as a function of time by fitting the Young−Laplace equation to the droplet profile yielding an average surface tension of 72.5±0.2 mN m −1 for water and 72.6±0.3 mN m −1 for water containing the nanoparticles ( Supplementary Fig. S2 ). Hence, the surface tension of the magnetic fluid was the same as that of pure water within the margin of error. Moreover, the surface tension of the magnetic fluid was time-independent, suggesting that the iron oxide nanoparticles did not have the tendency to migrate to the surface, as expected for electrostatically stabilized particles. Viscosity of the magnetic fluid The viscosities of pure Milli-Q water and Milli-Q water containing 0.2% (volume) of iron oxide nanoparticles were measured with a rheometer using a 50-mm cone-plate geometry with an angle of 2° (Paar Physica MCR 300 with CP 50-2). Measurements were done by varying the shear rate from 1 to 1,000 s −1 . The nominal viscosity values were calculated by averaging the viscosity between 10 and 100 s −1 . The viscosity of pure water was measured to be 0.97±0.02 mPa s and the viscosity of the magnetic fluid to be 1.01±0.02 mPa s ( Supplementary Fig. S2 ). The viscosity measurements were roughly in agreement with the Einstein model [46] . The Einstein model predicts that the relative increase in the viscosity due to the dispersed solids is 5 Φ /2, where Φ is the volume fraction of the solids. In our case 5 Φ /2=0.5%, underestimating somewhat the experimentally observed difference of 4%. An additional component to the viscosity is due to the alignment of the magnetic nanoparticles in an external magnetic field, which yields a contribution of 3 Φ /2 at maximum [47] , [48] according to the Hall−Busenberg model [49] , corresponding to 0.3% in our fluid. Such a small field-dependent contribution to the viscosity can be considered negligible in our measurements. Fabrication of superhydrophobic surface 1 Fluorinated Ag-coated Cu substrates were prepared as described in the literature [2] . AgNO 3 (99%, Fluka), 1 H ,1 H ,2 H ,2 H -perfluorodecanethiol (97%, Aldrich) and 1,2-dichloromethane (99%, Aldrich) were used as obtained. First, a mechanically polished copper substrate was coated with silver by immersing it into aqueous AgNO 3 solution (0.01 M) for 60 s, washing it with Milli-Q water and drying under nitrogen flow. Subsequently, the substrate was immersed into a solution of 1 H ,1 H ,2 H ,2 H -perfluorodecanethiol in 1,2-dichloromethane (0.001 M) for 10 min and washed afterwards twice with fresh 1,2-dichloromethane and dried under ambient conditions for few minutes. Fabrication of superhydrophobic surface 2 Silicone nanofilaments coated with fluorosurfactant were prepared as described in the literature with small modifications [50] . The nanofilaments were synthesized in an in-house-built gas-phase reactor operating under vacuum (ca. 0.1 mbar) at room temperature. Test-grade silicon (100) wafers were cleaned with an alkaline detergent (Deconex 11 Universal), rinsed thoroughly, dried, activated in H 2 /O 2 plasma (Gatan Solarus Model 950) and placed in the gas-phase reactor. Deionized water and methyltrichlorosilane (99%, Aldrich) were sequentially evaporated into the vacuum from separate lines controlled by Teflon valves. Finally the chamber was flushed with dry nitrogen. The nanofilament-coated substrate was then activated in O 2 /H 2 plasma and fluorinated with tridecafluorotetrahydro-octyltrichlorosilane (97%, ABCR). The latter reaction was done in an atmospheric reactor vessel flushed with dry nitrogen. The fluorosurfactant was injected into the reactor through a silicone septum, where it evaporated and reacted with the surface of the nanofilaments. Fabrication of superhydrophobic surface 3 Silicone nanofilament surfaces were prepared as described in the literature [50] . Cleaning of silicon (100) substrates was done as with Surface 2. Synthesis of the nanofilaments was done in an in-house built gas-phase reactor operating at atmospheric pressure. The reactor was purged with dry argon followed by pre-humidified argon until the relative humidity reached ca . 30%. The reactor was then sealed and methyltrichlorosilane injected through a silicone septum. Methyltrichlorosilane evaporated rapidly and nanofilaments were grown onto the surface. After ca . 1 h the reactor was purged with argon to stop the reaction and to remove the byproducts of gaseous reaction. Free-decay oscillations in a static magnetic potential well The oscillations of the magnetic droplets in a harmonic magnetic potential well were investigated using a high-speed camera (Casio EX-FH25). The measurements were carried out with three magnets (K&J Magnetics, NdFeB N52) with different sizes ( Supplementary Fig. S1 ). The magnets were positioned underneath or above the superhydrophobic surface and the magnetic field was determined from the distance between the droplet and the magnet based on field profiles measured with a Hall sensor (Lakeshore 475 DSP Gaussmeter with HMMT-6J02-VF probe). Measurements were performed with various separations between the magnet and the substrate to achieve different normal forces. In a typical experiment, the droplet was pipetted on the superhydrophobic surface away from the axis of the magnet and kept in place with a small (diameter 9 mm and height 4.5 mm) auxiliary magnet under the surface. With the help of the auxiliary magnet, the droplet was moved to 2.0±0.1 cm distance from the magnet axis and released by pulling the auxiliary magnet vertically away from the surface. The magnetic gradient from the main magnet then pulled the droplet towards the axis of the magnet. The resulting oscillatory motion was recorded with a high-speed camera at 1,000 fps. The auxiliary magnet allowed the droplet to be placed accurately to the distance of 2 cm from the main magnet before releasing it. In addition, the release of the droplet was gentle with the auxiliary magnet, which prevented the vertical bouncing of the droplet that was observed when the droplet was released directly from the pipette. Externally driven resonant measurements The forced oscillations were studied similarly as the free oscillations, with the exception that the magnet was attached to a linear precision positioning stage (Aerotech PRO165LM). The stage was controlled with a computer to produce sinusoidal linear oscillations with predefined amplitudes and frequencies f leading to a time-varying external field . The response of the droplet placed on a superhydrophobic surface above the stage and the magnet was observed with a high-speed camera as in the free oscillations and the amplitude of the oscillation was extracted from the videos. In frequency sweep measurements, was measured as a function of f and fitted with theoretical prediction calculated numerically with a custom Matlab script. Data analysis High-speed videos were analysed frame by frame with a custom Matlab script extracting the position of the droplet as a function of time. The external forces on the droplet were calculated from the droplet’s energy in the magnetic and gravitational fields, given by which can be approximated as where μ 0 is the permeability of vacuum, V the droplet volume, H the average internal magnetic field within the droplet (sum of the external field and the demagnetizing field of a spherical droplet), M the magnetization due to the average internal magnetic field and g the gravitational acceleration. When the distance between the axis of the cylindrical permanent magnet and the droplet is small (ca. less than half of the magnet radius), the magnetic field is approximately parabolic. The corresponding horizontal and vertical forces are given by Equation (3): In this approximation the position of the droplet as a function of time can be fitted with the solution of the general harmonic oscillator [32] , given piecewise for each half-oscillation n as where where A 0 is the starting amplitude, ω the angular frequency of the oscillation, the dimensionless sliding friction and the dimensionless viscous dissipation coefficient. Fitting with Matlab yields the desired parameters and . How to cite this article: Timonen, J. V. I. et al. Free-decay and resonant methods for investigating the fundamental limit of superhydrophobicity. Nat. Commun. 4:2398 doi: 10.1038/ncomms3398 (2013).